Nanomedicines reveal how PBOV1 promotes hepatocellular carcinoma for effective gene therapy There exists an urgent medical demand at present to develop therapeutic strategies which can improve the treatment outcome of hepatocellular carcinoma (HCC). Here, we explore the biological functions and clinical significance of PBOV1 in HCC in order to push forward the diagnosis and treatment of HCC. Using theranostical nanomedicines, PBOV1 is verified to be a key oncogene which greatly promotes HCC proliferation, epithelial-to-mesenchymal transition, and stemness by activating the Wnt/β-catenin signaling pathway. Therefore, single-chain antibody for epidermal growth factor receptor (scAb-EGFR)-targeted nanomedicine effectively silencing the PBOV1 gene exhibits potent anticancer effects. In vivo HCC-targeting siRNA delivery mediated by the theranostical nanomedicine remarkably inhibits the tumor growth and metastasis. In addition, the superparamagnetic iron oxide nanocrystals (SPION)-encapsulated nanomedicines possess high MRI detection sensitivity, which endows them with the potential for MRI diagnosis of HCC. This study shows that PBOV1 represents a prognostic biomarker and therapeutic target for HCC. Nowadays, there still exists an urgent medical demand to explore pharmacotherapeutic strategies that can improve the treatment outcome of hepatocellular carcinoma (HCC) [1] . Development of more potent drugs and therapeutic formulations relies on a better understanding about the mechanisms of HCC initiation and progression. Previous studies have shown that cancer stem cells (CSCs) capable of self-renewal and long-term repopulation [2] are decisive to local and distant tumor recurrence, and an effective suppression of this crucial population of cells is vital for improving the therapeutic outcome of HCC [3] . However, the molecular mechanisms for CSCs regulation remain largely unknown yet [4] . On the other hand, the role of epithelial-to-mesenchymal transition (EMT) in the advancement of HCC was gaining increasing attention in recent years. This multistep reprograming process of cellular state depends on the acquisition of stem cell-like attributes in tumors. Moreover, CSCs mediate tumor metastasis by maintaining their plasticity of transition between epithelial and mesenchymal states [5] . Prostate and breast cancer overexpressed 1 (PBOV1) is a human protein-coding gene with a 2501 bp single-exon mRNA, which is significantly overexpressed in several cancers, but not expressed in normal tissues. For example, it has been found to overexpress in the glandular epithelium of both primary and metastatic prostate cancer [6] . Samusik et al. [7] demonstrated the high levels of PBOV1 expression in breast cancer. Although these studies provide preliminary in vitro results that PBOV1 overexpression promoted cancer cell proliferation, its effect on EMT and CSCs regulation has not been reported. Interestingly, PBOV1 gene locates on chromosome 6 at 6q23–24, and genomic alterations of 6q23–24 associating with tumorigenesis and the progression of HCC have been affirmed in previous studies [8] , [9] . Unfortunately, the potential oncogenic role of PBOV1 in HCC initiation and progression remains almost unknown yet. In recent years, delivery of nucleic acids with polymeric nanocarriers has gained tremendous attention in cancer therapy. The nucleic acids loaded into nanocarriers can be protected against nuclease degradation in vivo [10] . Incorporation of superparamagnetic iron oxide nanocrystals (SPION) makes nanomedicines visible under magnetic resonance imaging (MRI), which simplifies the evaluation of pharmacokinetics and treatment outcome [11] . Furthermore, surface attachment of specific ligands recognizing molecular biomarkers on cancer cytomembrane (e.g., folate [12] and antibodies [13] ) may improve tumor-targeted drug delivery of nanomedicines both in vitro and in vivo [14] . Notably, epidermal growth factor receptor (EGFR), which belongs to the HER-erbB family of tyrosine kinase receptors, is overexpressed in many epithelial tumors as a cell transmembrane glycoprotein [15] , [16] . To date, anti-EGFR monoclonal antibodies such as cetuximab and panitumumab have been successfully applied alone or in combination with chemotherapeutic agents for cancer treatment in clinic, which implies that EGFR antibodies could be potent ligands directing drug delivery of nanocarriers to epithelial tumors including HCC [17] , [18] . In the present study, a HCC-targeting and MRI-visible nonviral carrier, EGFR single-chain antibody-modified graft copolymer of polyethylene glycol (PEG) and polyethylenimine (PEI) complexing SPION (abbreviated as scAb-EGFR-PEG-g-PEI-SPION), was developed to mediate effective nucleic acid delivery to HCC both in vitro and in vivo. Delivery of PBOV1 plasmid (PBOV1-pDNA) and PBOV1-siRNA plasmid (PBOV1-psiRNA) into HCC cells could up and downregulate the PBOV1 gene expression, respectively, upon which we hoped to understand whether and how PBOV1 expression levels affected the growth and metastasis of HCC. In addition, the potential of theranostical nanomedicine for treatment of HCC was explored. Identification of PBOV1 as a prognostic factor of human HCC The clue of PBOV1's oncogenic role in HCC came from the clinic. Comparison of the PBOV1 expression levels between the tumor tissues and adjacent nontumor tissues (ANT) of the same HCC patients strongly correlated the PBOV1 overexpression with oncogenesis in HCC patients. In other words, tumor tissues exhibited obviously higher PBOV1 expression at protein levels as compared with the paired ANT tissues according to immunohistochemistry (IHC) assay (Fig. 1a ). Similar results were also obtained for these clinical HCC samples in the western blotting and RT-PCR assays (Fig. 1b , Supplementary Fig. 1a ). Moreover, the overexpression level was found to affect the survival rates of HCC patients. 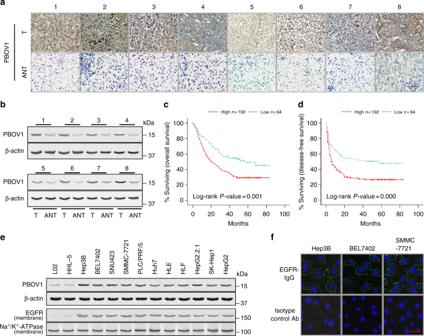Fig. 1 Clues of elevated expressions of PBOV1 and EGFR in HCC clinical specimens and cell lines.aImmunohistochemical stain (IHC) analysis of prostate and breast cancer overexpressed 1 (PBOV1) protein expression in each of the hepatocellular carcinoma (HCC) tissues (T) and adjacent nontumor tissue liver tissues (ANT) paired from the same patient. Scale bar, 100 μm.bWestern blotting analysis of PBOV1 protein expression in HCC tissues and paired ANT liver tissues from the same patient.cOverall survival of HCC patients with low PBOV1 expression versus patients with high PBOV1 expression (n= 286,P< 0.05, log-rank).dDisease-free survival of HCC patients with low PBOV1 expression versus patients with high PBOV1 expression (n= 286,P< 0.05, log-rank).eExpressions of PBOV1 and epidermal growth factor receptor (EGFR) determined by western blotting in the human normal hepatocyte cell lines (L02, HHL-5) and multiple HCC cell lines (Hep3B, BEL7402, SNU423, SMMC-7721, PLC/PRF/5, Huh7, HLE, HLF, HepG2.2.1, SK-Hep1, and HepG2).fConfocal laser scanning microscopy (CLSM) imaging of Hep3B, BEL7402, and SMMC-7721 cells via EGFR immunofluorescence staining with EGFR-IgG antibody or Isotype control antibody. Scale bar, 10 μm. (Blue, DAPI-indicating nuclei; Green, FITC indicating EGFR primary antibody aggregation). (See also Supplementary Fig.1) For 67.13% of patients (192/286) with high PBOV1 expression levels above the cutoff value of 3.5, tumor size, tumor number, and vascular invasion increased statistically as compared to patients with PBOV1 protein expression below the cutoff value (Supplementary Table 1 ). These patients also showed significantly poorer overall survival and disease-free survival (Fig. 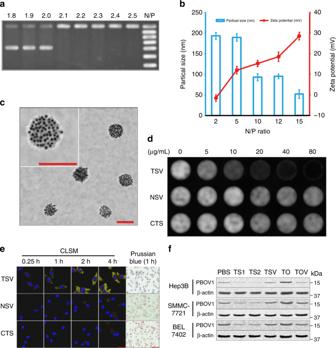Fig. 2 Physicochemical properties and HCC cell transfection of scAb-EGFR-targeted nanomedicine.aDetermination of plasmid DNA (pDNA) complexation at various nitrogen/phosphorus (N/P) ratios by gel retardation assay. Full complexation with single-chain antibody (scAb)-EGFR-PEG-g-PEI-SPION prevents DNA migration into the gel.bParticle size and zeta potential of scAb-EGFR-PEG-g-PEI-SPION/pDNA at various N/P ratios. Data were represented as means ± S.D. Error bars represent the S.D. values (n= 3).cTransmission electron microscopy (TEM) images of nanomedicine scAb-EGFR-PEG-g-PEI-SPION/pDNA. The gray halo around the dark SPION cluster indicates a polymeric shell. Scale bar, 100 nm.dT2-weighted magnetic resonance imaging (MRI) examination of different groups of Hep3B cells after 1 h of incubation at Fe concentrations of 0, 5, 10, 20, 40, and 80 μg/mL.eLeft four panels, confocal laser scanning microscopic (CLSM) imaging of different groups of Hep3B cells incubated for 0.25, 1, 2, 4 h, respectively, at Fe concentration of 20 μg/mL. Scale bar, 10 μm. (Blue, DAPI-indicating nuclei; red, POPO-3 indicating pDNA; green, Oregon Green 488-indicating delivery agent; Overlapping of red and green fluorescence to generate a yellow one, see also Supplementary Fig.1d). Right panel, Prussian blue staining images of different groups of Hep3B cells incubated at the same conditions as in CLSM studies. Scale bar, 50 μm. (Blue, indicating Fe aggregation; red, indicating nuclei).fProtein expression levels of PBOV1 in Hep3B, SMMC-7721, and BEL7402 cells relative to β-actin as control determined by western blotting assay 1c, d , Supplementary Table 2 ). Finally, reverse transcriptase polymerase chain reaction (RT-PCR) and western blotting analyses showed that PBOV1 mRNA and protein levels were markedly upregulated in multiple HCC cell lines including Hep3B, BEL7402, SNU423, SMMC-7721, PLC/PRF/5, Huh7, HLE, HLF, HepG2.2.1, SK-Hep1, and HepG2, as compared with human normal hepatocyte cell lines (L02 and HHL-5) (Fig. 1e , Supplementary Fig. 1b ). Taken together, PBOV1 expression might be a meaningful prognostic factor of HCC, which could influence oncogenesis and patient survival (Supplementary Table 2 ). Fig. 1 Clues of elevated expressions of PBOV1 and EGFR in HCC clinical specimens and cell lines. a Immunohistochemical stain (IHC) analysis of prostate and breast cancer overexpressed 1 (PBOV1) protein expression in each of the hepatocellular carcinoma (HCC) tissues (T) and adjacent nontumor tissue liver tissues (ANT) paired from the same patient. Scale bar, 100 μm. b Western blotting analysis of PBOV1 protein expression in HCC tissues and paired ANT liver tissues from the same patient. c Overall survival of HCC patients with low PBOV1 expression versus patients with high PBOV1 expression ( n = 286, P < 0.05, log-rank). d Disease-free survival of HCC patients with low PBOV1 expression versus patients with high PBOV1 expression ( n = 286, P < 0.05, log-rank). e Expressions of PBOV1 and epidermal growth factor receptor (EGFR) determined by western blotting in the human normal hepatocyte cell lines (L02, HHL-5) and multiple HCC cell lines (Hep3B, BEL7402, SNU423, SMMC-7721, PLC/PRF/5, Huh7, HLE, HLF, HepG2.2.1, SK-Hep1, and HepG2). f Confocal laser scanning microscopy (CLSM) imaging of Hep3B, BEL7402, and SMMC-7721 cells via EGFR immunofluorescence staining with EGFR-IgG antibody or Isotype control antibody. Scale bar, 10 μm. (Blue, DAPI-indicating nuclei; Green, FITC indicating EGFR primary antibody aggregation). (See also Supplementary Fig. 1 ) Full size image Nanocarriers for HCC-targeting nucleic acid delivery The MRI-visible nucleic acid nanocarriers incorporating 6-nm SPION, i.e., scAb-EGFR-PEG-g-PEI-SPION and nontargeted PEG-g-PEI-SPION, were prepared to deliver plasmids of DNA and siRNAs (PBOV1-pDNA, PBOV1-psiRNA1, and PBOV1-psiRNA2). The DNA and siRNAs were both used in the form of plasmids in order to achieve nanomedicines with comparable physical structures. The scAb-EGFR-targeted and MRI-visible nanocarrier (scAb-EGFR-PEG-g-PEI-SPION) measured 53 nm on average at room temperature in aqueous solution, as determined by dynamic light scattering (DLS) measurement. As demonstrated by numerous studies, the EGFR is known to be overexpressed on the membrane of many malignant cancer cells including HCC cells, which provided the basis for molecular therapies of HCC using EGFR inhibitors gefitinib, erlotinib, cetuximab, and antiangiogenic compounds (e.g., bevacizumab and sunitinib) [19] , [20] . Therefore, we assumed that EGFR antibody might also be an ideal candidate to mediate the HCC-targeting delivery of nanomedicines. In comparison with that in normal human hepatic cell lines (L02 and HHL-5), the EGFR expression levels were markedly upregulated in multiple HCC cell membranes, including Hep3B, BEL7402, SNU423, SMMC-7721, PLC/PRF/5, Huh7, HLE, HLF, HepG2.2.1, SK-Hep1, and HepG2 (Fig. 1e , Supplementary Fig. 1b ). Immunofluorescence assay also showed that the expression levels of EGFR protein on the membranes of Hep3B, BEL7402, and SMMC-7721 cells were high (Fig. 1f , Supplementary Fig. 1c ). Based on these results, scAb-EGFR as a HCC cell-specific ligand was conjugated to the distal ends of PEG chains, producing the final HCC-targeting nanocarrier scAb-EGFR-PEG-g-PEI-SPION. Agarose gel electrophoresis showed that the MRI-visible nanocarriers (scAb-EGFR-PEG-g-PEI-SPION and nontargeted PEG-g-PEI-SPION) efficiently complexed pDNA at appropriate nitrogen/phosphorus (N/P) ratios. Above N/P 2.1, complete retardation of pDNA motion was observed, indicating full pDNA complexation (Fig. 2a ). The final MRI-visible nanomedicine complexing pDNA was measured around 93 nm and +15.22 mV at N/P 10 (Fig. 2b ), with uniform spherical morphology and encapsulation of about 60 SPION in each nanomedicine particle according to the transmission electron microscopy observation (Fig. 2c ). We considered this nanomedicine size and zeta potential to be favorable for intravenous application and cell endocytosis. Moverover, SPION clustering inside nanomedicines has been demonstrated to significantly increase the MRI sensitivity, which is essential for in vivo applications [21] . Fig. 2 Physicochemical properties and HCC cell transfection of scAb-EGFR-targeted nanomedicine. a Determination of plasmid DNA (pDNA) complexation at various nitrogen/phosphorus (N/P) ratios by gel retardation assay. Full complexation with single-chain antibody (scAb)-EGFR-PEG-g-PEI-SPION prevents DNA migration into the gel. b Particle size and zeta potential of scAb-EGFR-PEG-g-PEI-SPION/pDNA at various N/P ratios. Data were represented as means ± S.D. Error bars represent the S.D. values ( n = 3). c Transmission electron microscopy (TEM) images of nanomedicine scAb-EGFR-PEG-g-PEI-SPION/pDNA. The gray halo around the dark SPION cluster indicates a polymeric shell. Scale bar, 100 nm. d T2-weighted magnetic resonance imaging (MRI) examination of different groups of Hep3B cells after 1 h of incubation at Fe concentrations of 0, 5, 10, 20, 40, and 80 μg/mL. e Left four panels, confocal laser scanning microscopic (CLSM) imaging of different groups of Hep3B cells incubated for 0.25, 1, 2, 4 h, respectively, at Fe concentration of 20 μg/mL. Scale bar, 10 μm. (Blue, DAPI-indicating nuclei; red, POPO-3 indicating pDNA; green, Oregon Green 488-indicating delivery agent; Overlapping of red and green fluorescence to generate a yellow one, see also Supplementary Fig. 1d ). Right panel, Prussian blue staining images of different groups of Hep3B cells incubated at the same conditions as in CLSM studies. Scale bar, 50 μm. (Blue, indicating Fe aggregation; red, indicating nuclei). f Protein expression levels of PBOV1 in Hep3B, SMMC-7721, and BEL7402 cells relative to β-actin as control determined by western blotting assay Full size image Internalization of targeted nanomedicines into HCC cells It is well-known that MRI can be used as a noninvasive tool to monitor drug delivery if the nanomedicines are MRI visible. Thus, the effect of HCC-targeting on the cellular uptake of SPION-containing nanomedicines was evaluated by MRI scanning. When Fe concentration in the cell culture medium increased from 5 to 80 μg/mL, the MRI T2-weighed signal intensity in Hep3B cells receiving scAb-EGFR-PEG-g-PEI-SPION/psiRNA-vector (TSV group) decreased much more significantly than that in the cells receiving nontargeted PEG-g-PEI-SPION/psiRNA-vector (NSV group). However, when excessive free EGFR antibody was present in the culture medium, the MRI T2-weighed signal intensities in cells receiving scAb-EGFR-targeted nanomedicine (CTS group) turned back to similar levels as detected in the NSV group (Fig. 2d ). The confocal laser scanning microscopic (CLSM) observation of the Hep3B cells incubated with multiple fluorescence-labeled nanomedicines obtained consistent data. At all investigated cell incubation time (0.25, 1, 2, and 4 h), the targeted nanomedicine (TSV group) was much more effectively taken up by the cells than the nontargeted nanomedicine (NSV group), according to the strong green (indicating delivery agent) and red (indicating plasmid) fluorescence overlapping in the cell membrane and cytoplasm. The nontargeted nanomedicine (NSV group) only showed strong blue fluorescence indicating nuclei. Preincubation of Hep3B cells with free EGFR antibody (CTS group) significantly inhibited the EGFR-mediated cell uptake of the scAb-EGFR-targeted nanomedicine. Moreover, CLSM imaging showed the internalization process of the scAb-EGFR-targeted nanomedicine into Hep3B cells. That is, it was first bound to the cell membrane (0.25 h) and then gradually entered into the cells (1 h) until getting a saturated intracellular concentration (2 h vs. 4 h) (Fig. 2e , Supplementary Fig. 1d ). Prussian blue staining showed different iron depositions inside various Hep3B cells, which accorded well with the MRI and CLSM analysis results. That is, most of the cells in the TSV group showed strong blue staining owing to the EGFR-mediated high level of nanomedicine uptake, whereas only few cells in the NSV and CTS groups showed weak blue staining, indicating very low level of SPION uptake due to the absence of EGFR-targeting function of nanomedicine (Fig. 2e ). Obviously, the EGFR membrane proteins of Hep3B cells can mediate highly efficient internalization of the MRI-visible nanomedicine scAb-EGFR-PEG-g-PEI-SPION. PBOV1 promotes growth and metastasis of HCC cells in vitro The abilities of scAb-EGFR-PEG-g-PEI-SPION/PBOV1-pDNA (for TO group) to effectively upregulate, whereas scAb-EGFR-PEG-g-PEI-SPION/PBOV1-psiRNA (for TS1 and TS2 groups) to effectively downregulate the PBOV1 protein expression were validated in Hep3B, SMMC-7721, and BEL7402 HCC cell lines. As shown in Fig. 2f and Supplementary Figs. 2 and 4 , compared with the three control groups (phosphate buffered saline (PBS), TSV, and TOV), the TO group showed much higher, whereas the TS1/TS2 groups showed much lower PBOV1 expression level. In order to further understand the oncogenic functions of PBOV1, the effects of the up and downregulated PBOV1 expressions on HCC proliferation, invasion, and migration were investigated in Hep3B cells, as a representative HCC cell line. PBOV1 expression obviously affected HCC cell proliferation (Fig. 3a ). The proportions of G2/M and S-phase cells were significantly increased and meanwhile, the expression of cell cycle marker cyclin D1 was markedly upregulated due to the PBOV1 overexpression in the TO group. In contrast, the proportions of G2/M and S-phase cells were significantly decreased and expression of cyclin D1 was obviously downregulated due to the PBOV1 gene silencing in the TS1 and TS2 groups (Fig. 3b, d , Supplementary Fig. 5c ). Meanwhile, the anchorage-independent growth and colony formation abilities (number and size) of Hep3B cells were significantly increased via PBOV1 upregulation, whereas they were decreased remarkably following PBOV1 silencing (Fig. 3c ). Moreover, as determined by the terminal deoxynucleotidyl transferase-mediated dUTP nick end labeling assay (TUNEL) assay, PBOV1 upregulation in the TO group resulted in obviously decreased cell apoptosis and lower expression of apoptotic marker cleaved-caspase 3, whereas PBOV1 silencing in the TS1 and TS2 groups showed an opposite effect (Fig. 3c, d , Supplementary Fig. 5a ). Consequently, PBOV1 overexpression led to an obviously upregulated expression of proliferation marker (suvivin) and significantly increased growth rate of HCC cells, while PBOV1 silencing had an opposite effect (Fig. 3a, d , Supplementary Fig. 5c ). Fig. 3 The relationship between PBOV1 expression level and Hep3B cell growth/metastasis property in vitro. a Hep3B cell growth rates determined by MTT assay. b Hep3B cell cycle analysis by flow cytometry assay. c Cell proliferation reflected by anchorage-independent growth assay (first panel, top down; Scale bar, 1 mm), cell colony formation assay (second panel, top down; Scale bar, 10 mm), and terminal deoxynucleotidyl transferase-mediated dUTP nick end labeling assay (TUNEL) cell apoptosis assay (third panel, top down; Scale bar, 20 μm) (assay; Blue, DAPI-indicating nuclei; green, FITC indicating apoptotic nuclei). d Protein expression levels of survivin, cyclin D1, and cleaved-caspase 3 determined by western blotting assay. e Tube formation assay by human liver tumor endothelial cells (SK-Hep1) cultured on Matrigel-coated plates with conditioned media collected from the Hep3B cell incubation (first panel, top down; Scale bar, 100 μm). Hep3B cell migration ability determined by transwell migration assay (second panel, top down; Scale bar, 50 μm). Hep3B cell invasion ability determined by transwell invasion assay (third panel, top down; Scale bar, 50 μm). Hep3B cell mobility measured by testing the rate of wound healing at 24 h after serum starvation and wound creation (fourth panel, top down; Scale bar, 500 μm) (See also Supplementary Fig. 5b ). f Protein expression levels of angiogenesis marker HIF-1α, epithelial markers α-Catenin and E-cadherin, and mesenchymal markers N-cadherin and Vimentin determined by western blotting assay. g Immunofluorescence assays for epithelial markers α-Catenin and E-cadherin, and mesenchymal markers N-cadherin and Vimentin. Scale bar, 20 μm (Blue, DAPI-indicating nuclei; green, FITC indicating α-Catenin or N-cadherin protein; red, Cy5 indicating E-cadherin or Vimentin protein). (See also Supplementary Fig. 5d ). Data were represented as means ± S.D. Error bars represent the S.D. values ( n = 3; * P < 0.05; ns, not significant. Significant differences were analyzed by two-way ANOVA with multiple comparisons for ( a ); Student’s t test for ( a ) and ( b ), compared with PBS control group) Full size image When the Hep3B, SMMC-7721, and BEL7402 HCC cells were transfected with nontargeted nanomedicines in the same plasmid concentrations, the PBOV1 expression level was almost unchanged in the NS1, NS2, and NO groups both in vitro and in vivo due to the minimal cell uptake of the nontargeted nanomedicines (Supplementary Figs. 2a, c , 3c , 4c ). Consequently, cell proliferation abilities were nearly unaffected, as revealed by the MTT assay in vitro and analysis of orthotropic tumor growth in vivo (Supplementary Figs. 2b, d , 3d , and 4d ). These results verified the critical role of targeting delivery in nanocarrier-mediated regulation of gene expression in HCC, and also excluded the possibility of the nanocarrier to affect hepatoma cell proliferation. The effects of PBOV1 expression levels on the metastatic potentials of HCC cells were investigated in Hep3B cells as an example. First, the tube formation assay was conducted to test the angiogenic potential of human hepotoma endothelial cells (SK-Hep1), which had been activated by the Hep3B cell-secreted angiogenic factors [22] . HIF-1α, which is known as a major transcriptional factor regulating angiogenesis and vascular permeability through inducing proangiogenic genes (e.g., VEGF) and glycolytic enzymes, has been found to be consistently upregulated in various cancers including HCC, and associated with poor clinical outcomes in patients [23] , [24] . An increased nuclear translocalization of HIF-1α can promote tube formation and VEGF secretion in endothelial cells [25] , and HIF-1α has been found to be vital in stem cell maintenance via the Wnt/β-catenin pathway [26] . As PBOV1 upregulation increased the expression of angiogenic marker HIF-1α in Hep3B cells, endothelial cell culture with the medium collected from Hep3B cell incubation resulted in most tube formation in the TO group. On the contrary, as PBOV1 silencing decreased the expression of HIF-1α in Hep3B cells, endothelial cell culture with the medium collected from Hep3B cell incubation resulted in least tube formation in the TS1 and TS2 groups (Fig. 3e, f , Supplementary Fig. 5d ). Then, the Boyden chamber migration assay and the Boyden chamber invasion assay were performed to detect the effect of PBOV1 expression on the Hep3B cell migration and invasion potential, respectively. As shown in Fig. 3e , in the Boyden chamber migration assay, the cells with PBOV1 upregulation migrated vigorously through a noncoating porous membrane, leading to the largest number of cells residing at the filter bottom (TO group). In contrast, the PBOV1-downregulated cells exhibited least cells residing at the filter bottom due to poorest migration (TS1 and TS2 groups). Boyden chamber invasion assay obtained consistent results. In other words, cells in the TO group penetrate the basement membrane-mimicking Matirgel most effectively, leading to increased number of invasion cells at the filter bottom. However, cells in the TS1 and TS2 groups behaved exactly the other way around (Fig. 3e ). In addition, in the wound-healing assay, cells in the TO group migrated most effectively, leading to the narrowest wound gaps at both 12- and 24-h incubation after serum starvation and wound creation. On the contrary, the TS1 and TS2 groups exhibited the poorest wound-healing performance (Fig. 3e , Supplementary Fig. 5b ). These results indicated that PBOV1 overexpression reinforces, whereas PBOV1 silencing suppresses the metastasis potential of Hep3B cells. EMT process has been proposed as a critical mechanism during cancer progression and metastasis [27] . EMT, which loosens cell–cell adherence to endow the cells with enhanced migratory and invasive properties, can be adopted by tumors to increase invasiveness and stem-like features during metastatic progression [28] . Especially, EMT may be induced in a subset of metastatic CSCs, depending on which the population becomes highly aggressive and can spread in the body [27] . Therefore, the EMT pathway could be targeted to prevent metastasis, which represents a strategy for cancer treatments [29] . Unfortunately, the drugs specifically designed for EMT reversal are not available nowadays. The expressions of EMT markers were determined to explore whether the PBOV1 expression-dependent metastasis potentials of HCC were owing to the EMT process. Compared with the PBS control group, the TO group with PBOV1 overexpression showed the significantly downregulated epithelial marker's (α-Catenin and E-cadherin) expression, whereas the much upregulated mesenchymal marker's (N-cadherin and Vimentin) expression in Hep3B cells. However, the TS1 and TS2 groups with PBOV1 silencing showed the obviously upregulated α-Catenin and E-cadherin expressions, whereas the remarkably downregulated N-cadherin and Vimentin expressions in Hep3B cells (Fig. 3f , Supplementary Fig. 5d ). Immunofluorescence assays also confirmed that the expressions of epithelial markers (α-Catenin and E-cadherin) were significantly downregulated, whereas the expressions of mesenchymal markers (N-cadherin and Vimentin) were significantly upregulated in the PBOV1-upregulated Hep3B cells (TO group). Hep3B cells in TS1 and TS2 groups with PBOV1 gene silencing exhibited the opposite trend of EMT marker expressions (Fig. 3g ). In addition, in line with the results of growth and metastasis assays, the TSV, TOV, and PBS control groups without PBOV1 regulation showed no difference in the expression levels of growth markers and metastasis markers (Fig. 3d, f, g , Supplementary Fig. 5c, d ). Apparently, the PBOV1 gene promoted HCC metastasis via regulating the EMT process. These results also evidenced that the scAb-EGFR-targeted nanocarrier incorporating PBOV1-siRNA possessed the potential to act as an effective nanomedicine in suppressing the EMT process. Taken together, when PBOV1 overexpression was established in the TO group, growth and metastasis of HCC cells was promoted as compared with that in the PBS, TSV, and TOV groups. In contrast, when the HCC cells were incubated with scAb-EGFR-PEG-g-PEI-SPION/PBOV1-psiRNA1 and scAb-EGFR-PEG-g-PEI-SPION/PBOV1-psiRNA2 (TS1 and TS2 groups), the growth and metastasis significantly decreased, following the downregulation of PBOV1 gene expression. In vivo tumor detection with HCC-targeting nanomedicine Tumor area accumulation of the scAb-EGFR-targeted nanomedicines simultaneously labeled with MRI T2 contrast agent SPION and near-infrared fluorescence (NIRF) agent Alexa Fluor 750 in liver orthotropic HCC mice models was monitored by MRI and NIRF bimodal imaging. MRI T2 imaging showed that the tumor area became hypointense from 0.5 to 24 h after injection of scAb-EGFR-targeted nanomedicine, reaching the lowest signal intensity at 2 h after injection (TSV group). However, tumor area in mice receiving the nontargeted nanomedicine showed much less decrease in MRI T2 signal intensity (NSV group) (Fig. 4a ). In vivo NIRF imaging of mice at various postinjection time points from 0 to 24 h obtained consistent results showing different tumor accumulation behaviors of the Alexa Fluor 750-labeled scAb-EGFR-targeted nanomedicine (TSV) and nontargeted nanomedicine (NSV group) administered via the tail vein (Fig. 4b , Supplementary Fig. 10 ). Prussian blue staining for iron deposition in tumor tissue was highly supportive of the MRI and NIRF imaging results. Compared to the NSV group, the TSV group exhibited much more blue stains for Fe depositions, indicating high level of SPION transported to tumor tissue by scAb-EGFR-targeted nanomedicine (Fig. 4c ). Fig. 4 In vivo biodistribution and toxicological study of theranostical nanomedicine in Hep3B liver orthotropic model. a T2-weighted MRI examination showing a nonlinear change in tumor signal intensity against tracing time (0, 0.5, 2, 6, 12, and 24 h after tail vein single injection). Yellow arrows indicate the location of the tumor. b Near-infrared fluorescence (NIRF) imaging of mice 2 h after nanomedicine single injection. The fluorescent reporter used for NIRF was Alexa Fluor 750. Yellow arrows indicate the location of the tumor (See also Supplementary Fig. 10 ). c Prussian blue staining performed on histological sections of orthotropic tumors 2 h after single injection. Scale bar, 100 μm. d NIRF images of various mice organs harvested 2 h after nanomedicine single injection (see also Supplementary Fig. 10 ). e Averaged fluorescence intensities of mice tumors and major organs at 2, 6, and 12 h after a single injection of nanomedicine. f Serum liver function markers alanine transaminase (ALT)/total bilirubin (TBIL) and renal function markers blood urea nitrogen (BUN)/creatinine (Cr) were assessed during the period from 0 to 20 days after namomedicine injection once a day under therapeutic dosage (plasmid dose 8 μg). g Haematoxylin and eosin (H&E) staining of the liver and kidney tissues from mice after 20 days of treatment for evaluations of tissue inflammation and structural damage. Scale bar, 20 μm. (nanomedicine injected once a day at plasmid dose 8 μg). h Schedule illustration of in vivo study. Data were represented as means ± S.D. Error bars represent the S.D. values ( n = 12, * P < 0.05, Student’s t test, compared with NSV group or PBS control group). Full size image Ex vivo fluorescence imaging of major organs (brain, lung, heart, liver, spleen, and kidney) and tumor excised from mice at different postinjection times (2, 6, and 12 h) was conducted to show the in vivo biodistribution of Alexa Fluor 750-labeled nanomedicine (TSV and NSV groups) injected via the tail vein. Both the scAb-EGFR-targeted nanomedicine (TSV) and nontargeted nanomedicine (NSV group) showed strong liver accumulation. In contrast, their accumulation in all other organs was very weak. More excitingly, the TVS group showed much stronger tumor fluorescence than the NSV group, indicating much better tumor accumulation via EGFR targeting (Fig. 4d, e ; Supplementary Fig. 10 ). Due to their leaky blood vessels, solid tumors possess significantly higher vascular permeability and hydraulic conductivity than normal ones, which is favorable for nanomedicine delivery to tumor tissues. As the pore sizes of blood vessels in the majority of solid tumors range from 380 to 780 nm [30] , our scAb-EGFR-targeted nanomedicines measuring around 100 nm can easily cross the tumor blood vessels. Moreover, the scAb-EGFR modification promotes cell uptake and tumor retention of nanomedicine through recognizing EGFR protein on the HCC cell membrane. Obviously, not only the passive tumor accumulation derived from the enhanced permeation and retention effect [31] , but also the scAb-EGFR-mediated active targeting contributed significantly to the remarkable tumor accumulation of HCC-targeting nanomedicines in the liver orthotropic HCC xenograft models. In vivo toxicity of theranostical nanomedicine After the tail vein injection of the scAb-EGFR-targeted nanomedicine, body weights of the animals, tissue inflammation and structural damage in liver and kidney, and serum biochemical data were analyzed. Serum biochemical tests included measurements of liver functional clinical biomarkers alanine transaminase (ALT)/total bilirubin (TBIL), and renal functional clinical biomarkers serum creatinine (Cr)/blood urea nitrogen (BUN). Under the in vivo therapeutic nanomedicine dosage over the 20 days of treatment, significant differences from the PBS control group were not observed in body weights for any of the nanomedicine injected groups (Supplementary Fig. 9c ). The TSV group (scAb-EGFR-PEG-g-PEI-SPION/psiRNA-vector) was employed as a representative nanomedicine to evaluate the liver and kidney toxicity during the treatment period. Although mild and self-limited elevations in ALT (from 3 to 12 days) and TBIL (12 to 20 days treatment time) were shown, no obvious changes in BUN and Cr levels were found in animals receiving injection once a day for 20 days (Fig. 4f ). Moreover, the histological analysis showed no obvious structural damage (e.g., necrosis or cellular cloudy swelling) in liver and kidney after nanomedicine treatment for 20 days (Fig. 4g, h ). These results demonstrated that administration of the theranostical nanomedicine only caused a transient liver functional abnormality, but did not lead to any substantial detrimental damage in the liver and kidney. In vivo HCC growth and metastasis promoted by PBOV1 The effect of PBOV1 expression on HCC growth in vivo was examined in liver orthotropic models using nude mice-bearing human Hep3B, SMMC-7721, and BEL7402 hepatoma, respectively (Fig. 5a, b ). The in vivo therapies began at day 11 after HCC cell transplantation and finished after 20 days of treatment (Fig. 4h ). Compared with the three control groups (PBS, TSV, and TOV) showing similar tumor weight (Fig. 5a ) and close PBOV1 expression levels (Fig. 5b ), the TO group showed significantly increased tumor weight accompanied with upregulated expressions of survivin (proliferation marker)/cyclin D1 (cell cycle marker) and downregulated expression of cleaved-caspase 3 (apoptotic marker) following PBOV1 overexpression, whereas the TS1 and TS2 groups showed obviously decreased tumor weight accompanied with downregulations of survivin/cyclin D1 and upregulation of cleaved-caspase 3 following PBOV1 silencing, according to western blotting and IHC assays (Fig. 5c–f ). Determination of tumor volume by MRI T2 scan also obtained consistent results to show the growth of orthotropic liver tumors (Fig. 5c, d ). Furthermore, immunofluorescence assay further showed that the fluorescence signals for proliferating markers (BrdU and Ki67) on the tissue sections of orthotropic tumors increased in the TO group, but decreased in the TS group (Fig. 5f ). Fig. 5 In vivo effects of nanomedicines on proliferation activities in HCC liver orthotropic and subcutaneous models. a Tumor weight measured at day 20 after treatment began in Hep3B, SMMC-7721 and BEL7402 liver orthotropic model. b Protein expression levels of PBOV1 determined by western blotting assay in Hep3B, SMMC-7721, and BEL7402 liver orthotropic tumor tissues from mice after treatment for 20 days. c Kinetic of the liver orthotropic tumor growth measured by MRI T2 scan at 2 h after nanomedicine injection (nanomedicines injected once every day from day 11; to visulaize the tumors of PBS group by MRI, TOV nanomedicine was injected 2 h before MRI scan). d First panel, MRI T2 scan for liver orthotropic tumors; second panel, optical imaging of liver showing orthotropic tumors at day 20 after treatment began. e Protein expression levels of proliferation marker survivin, cell cycle marker cyclin D1 and apoptotic marker cleaved-caspase 3 in Hep3B liver orthotropic tumor tissues at day 20 after treatment began. f First and second panel from top down, protein expressions of PBOV1 determined by IHC in liver orthotropic tumors in various treatment groups, and magnified view showing location of PBOV1 expression inside cancer cells (Scale bar, 50 μm); third and fourth panel from top down, in vivo tumor cell proliferation abilities measured by immunofluorescence staining assays for Bromodeoxyuridine (BrdU) and Ki67; fifth panel from top down, tumor apoptosis detected by TUNEL assay (Scale bar, 20 μm) (Blue, DAPI-indicating nuclei; red, Cy5 indicating BrdU location; green, FITC indicating Ki67 protien or apoptotic nuclei). g Observation of the tumor inhibition effect in subcutaneous tumor model during the 20 days of treatment (see also Supplementary Fig. 6 ). Data were represented as means ± S.D. Error bars represent the S.D. values ( n = 12; * P < 0.05; ns, not significant. Significant differences were analyzed by two-way ANOVA with multiple comparisons for c and g ; Student’s t test for ( a , c and g ), compared with PBS control group) Full size image As determined in TUNEL staining assay, PBOV1 upregulation led to decreased HCC apoptosis (TO group), whereas PBOV1 silencing functioned the other way around (TS1 and TS2 groups) (Fig. 5f , Supplementary Fig. 6a ). In addition, injection of nontargeted PEG-g-PEI-SPION/plasmids (NS1, NS2, and NO groups) did not obviously affect both the PBOV1 expression and tumor weight (Supplementary Fig. 2c, d ), most likely due to the insufficient cell uptake of nontargeted nanomedicines as already found in vitro (Supplementary Figs. 2a , 3c , and 4c ). Similar tumor growth trend was observed in the Hep3B subcutaneous tumor model (Fig. 5g ). In order to gain further insight into the effect of PBOV1 expression on HCC metastasis, pulmonary metastasis potential was investigated by determining the formation of lung metastatic nodules in nude mice receiving tail vein injection of human Hep3B cells (Fig. 6a ). After 20 days of treatment, the three control groups (PBS, TSV, and TOV) showed clear lung metastasis, and the upregulation of PBOV1 expression even resulted in many more lung metastatic nodules and meanwhile, much severer pulmonary edema due to tumor-associated inflammation (TO group). On the contrary, downregulation of PBOV1 expression resulted in significantly decreased number of lung metastatic nodules and meanwhile, minimum pulmonary edema (TS1 and TS2 groups) (Fig. 6a, b ). Microvessel density (MVD) staining assay showed that PBOV1 upregulation led to enhanced angiogenesis (TO group), whereas PBOV1 silencing functioned the other way around (TS1 and TS2 groups) (Fig. 6a , Supplementary Fig. 6b ). Fig. 6 In vivo effects of nanomedicines on metastasis and stemness activities. a Pulmonary metastasis (first panel, top down) and H&E staining (second panel, top down; Scale bar, 200 μm) of the metastatic tumor after 20 days of treatment; third panel from top down, tumor angiogenesis determined by microvessel density (MVD) assay (Scale bar, 20 μm; Blue, DAPI-indicating nuclei; green, FITC indicating CD31 protein). b Pulmonary metastatic tumor nodes counted after 20 days of treatment. c Protein expression levels of angiogenesis marker HIF-1α, epithelial markers α-Catenin and E-cadherin and mesenchymal markers N-cadherin and Vimentin in pulmonary metastasis tumor tissues. d First panel from top down, cell stemness measured by sphere formation assay (Scale bar, 100 μm); second panel from top down, proportions of cancer stem cells (CSCs) measured by Hoechst 33342 dye exclusion assay; third panel from top down, flow cytometry analyses of the percentage of CD133 + / EpCAM + cells in Hep3B cell populations; 4th panel from top down, in vivo CD133 + cancer stem cell propotion displayed by immunofluorescence staining (Scale bar, 20 μm; Blue, DAPI-indicating nuclei; green, FITC indicating CD133 protien location). e In vitro protein expression levels of general stem cell markers (OCT4, NANOG, c-myc) and cancer stem cell surface markers (CD133, EpCAM) determined by western blotting assay. f Effect of nanomedicine treatments on tumor incidence rates and growth speeds in subcutaneous tumor model established via subcutaneous injection of 1 × 10 4 Hep3B cells. g Oncogenic potential determined by limiting dilution assay to measure tumor incidence; various amounts of Hep3B cells (1 × 10 3 , 1 × 10 4 , 1 × 10 5 or 1 × 10 6 ) were injected subcutaneously before nanomedicine treatment (see also Supplementary Fig. 7 ). h Protein expression levels of stem cell markers and cancer stem cell surface markers in subcutaneous tumor tissues. Data were represented as means ± S.D. Error bars represent the S.D. values ( n = 12; * P < 0.05; ns, not significant. Significant differences were analyzed by two-way ANOVA with multiple comparisons for ( f ); Student’s t test for ( b ) and ( f ), compared with PBS control group) Full size image As shown in the western blotting assay (Fig. 6c ), the upregulated angiogenesis marker (HIF-1α) and mesenchymal markers (N-cadherin and Vimentin), but downregulated epithelial markers (α-Catenin and E-cadherin), were detected in the TO group, whereas the TS1 and TS2 groups behaved the other way around. These results demonstrated that PBOV1 promoted the metastasis of HCC in vivo through inducing the EMT process, which was in line with the in vitro results on migration and invasion of HCC (Fig. 3e–g ). HCC stemness regulated by HCC-targeting nanomedicine In Hep3B cells, upregulation of PBOV1 expression significantly promoted the sphere formation potential and increased the proportion of CSCs (TO group), whereas PBOV1 silencing obviously suppressed the sphere formation potential and decreased the proportion of CSCs (TS1 and TS2 groups). In contrast, cell transfection with scAb-EGFR-targeted nanomedicines carrying psiRNA and pDNA vectors had no obvious effect on the sphere formation potential and proportion of CSCs (TSV and TOV groups) (Fig. 6d ). Moreover, upregulation of PBOV1 expression resulted in high expression levels of stem cell markers (OCT4, NANOG, and c-myc) and CSC surface markers (CD133 and EpCAM) in the TO group, whereas downregulation of PBOV1 expression behaved oppositely (TS1 and TS2 groups) both in vitro and in vivo (Fig. 6d, e, h ). The above results revealed that the PBOV1 expression level is positively related to the stemness of HCC cells. Therefore, tumorigenicity of Hep3B HCC cells in vivo was obviously affected by the PBOV1 expression levels. In subcutaneous tumor models, elevating the stemness by PBOV1 overexpression induced obviously increased tumor incidence rate (TO group), whereas reducing the stemness by PBOV1 silencing led to much lowered tumor incidence rate (TS1 and TS2 groups) (Fig. 6f, g , Supplementary Fig. 7 ). For instance, when 1 × 10 4 Hep3B cells were injected, tumor was developed in 33%, 25%, and 25% of mice in the TSV, TOV and PBS groups, respectively. In contrast, tumor was formed in as many as 75% of mice in the TO group, whereas no tumor was developed in the TS1 and TS2 groups (Fig. 6f ). Moreover, for the injection at less cell number of 1 × 10 3 , only the TO group showed the ability to form tumor (still 25% tumor incidence) (Fig. 6f, g , Supplementary Fig. 7 ). The tumor growth rate was also found to be positively related to the PBOV1 expression levels, i.e., the higher the PBOV1 expression level the faster, the tumor growth at all cell injection numbers (Figs. 5c, g , 6f, g , Supplementary Fig. 7b ). PBOV1 activates β-catenin to promote tumor aggressiveness To explore the mechanism by which PBOV1 activates β-catenin signaling, affinity purification and mass spectrometry (MS) were used to identify PBOV1-interacting proteins. As shown in Fig. 7a, b , β-catenin was found as an interactor of PBOV1. Importantly, reciprocal coimmunoprecipitation and western blotting assays further validated that PBOV1 formed a complex with β-catenin (Fig. 7c ). Immunostaining analysis showed that PBOV1 and β-catenin co-localized in the nucleus (Fig. 7d ). Luciferase reporter assay showed that overexpression of PBOV1 enhanced, whereas knockdown PBOV1 impaired, the activity of β-catenin luciferase reporter (Fig. 7e ). Moreover, overexpression of PBOV1 increased total β-catenin expression and reduced phosphor-β-catenin (Ser33/37/Thr41) expression, and vice versa (Fig. 7f, g ). GSK-3β phosphorylates β-catenin at Ser33, Ser37, and Thr41 and destabilizes it, thus we reasoned that PBOV1 might protect β-catenin from phosphorylating by GSK-3β via impairing the interaction between GSK-3β and β-catenin. Indeed, overexpression of PBOV1 reduced the interaction between GSK-3β and β-catenin in a dose-dependent manner (Fig. 7h ). However, no interaction was noticed between PBOV1 and GSK-3β, which indicates that PBOV1 competes with GSK-3β for β-catenin binding. Immunostaining showed that PBOV1 enhanced accumulation of β-catenin in the nucleus (Fig. 7i ). Real-time PCR analysis proved that overexpression of PBOV1 promoted, while knockdown of PBOV1 inhibited the expression of β-catenin downstream genes (Fig. 7j ). Overall, these results revealed that PBOV1 activates β-catenin and subsequently promotes HCC aggressiveness and progression. Fig. 7 PBOV1 binds to β-catenin and activates Wnt/β-catenin signaling. a Representative picture of coomassie blue staining of proteins co-immunoprecipitated with PBOV1. b Representative MS plots and sequences of peptides from β-catenin. c Immunoprecipitation assay confirming interaction between PBOV1 and β-catenin. d Representative confocal images showing colocalization of PBOV1 and β-catenin (Scale bar, 10 μm). e β-catenin luciferase-reporter activities analyzed in various groups of Hep3B cells. Data were represented as means ± S.D. Error bars represent the S.D. values ( n = 3; * P < 0.05. Significant differences were analyzed by Student’s t test, compared with PBS control group). f Protein expression levels of β-catenin in the nuclear fraction and Phospho-β-catenin (Ser33/37/Thr41) in Hep3B cells in vitro determined by western blotting assay. P84 and β-actin served as loading control. g Protein expression levels of total β-catenin and Phospho-β-Catenin (Ser33/37/Thr41) in Hep3B subcutaneous tumor tissues determined by western blotting assay. h PBOV1 attenuates interactions between β-catenin and GSK-3β in dose-dependent manner. i Immunofluorescence staining of β-catenin in the indicated Hep3B cells. (Scale bar, 20 μm; Blue, DAPI-indicating nuclei; green, FITC indicating β-catenin protein). j Real-time PCR analysis demonstrating an apparent overlap between β-catenin-dependent gene expression and PBOV1-regulated gene expression. The pseudocolour represents the intensity scale for indicated treatment groups versus PBS control group, calculated by log 2 transformation Full size image In the past few years, compelling evidence has emerged to support the CSCs model for solid tumors, including HCC. Unfortunately, although >40% of HCCs are thought to arise from CSCs, the genetic basis for CSC formation and thereafter HCC proliferation and EMT remain poorly understood [32] . Therefore, identification of key functional oncogenes for CSC formation in HCC is important, since it could lead to efficient treatment strategies for this fatal disease [3] , [33] . On the other hand, PBOV1 has been found to significantly overexpress in several cancers, but not in normal tissues. Although previous studies provided preliminary results that PBOV1 overexpression promoted cancer cell proliferation [6] , its effect on EMT and CSCs regulations remained unclear [34] . Moreover, the oncogenic role of PBOV1 in HCC has not been reported at all. The present study explored the oncogenic role of PBOV1 in growth and metastasis of HCC by using a scAb-EGFR-targeted theranostical nanomedicine platform. To learn whether the expression level of a suspected oncogene is really related to tumor growth and metastasis, an effective regulation of its expression is crucial, which depends on the design of a powerful tool to transport nucleic acids including DNA and siRNA plasmids into cancer cells. Recently, plasmids were effectively complexed with nonviral nanocarrier based on diblock copolymer (PEG-g-PEI) and SPION, which led to the formation of MRI-visible nanomedicines for HCC oncogene identification and effective therapy [12] , [13] . Modification of nanomedicines with the scAb-EGFR significantly improved the efficiency of delivering nanomedicines into HCC cells overexpressing EGFR on cell membrane, based on which we not only identified PBOV1 as an important oncogene in HCC, but also revealed its molecular mechanisms to affect growth and metastasis of HCC. Wnt/β-catenin signaling has been well-demonstrated to play pivotal roles in promoting EMT and stemness of cancer cells and subsequently metastasis [35] , [36] , [37] . In this study, we find that PBOV1 binds to β-catenin to protect it from phosphorylating by GSK-3β and thus activates Wnt/β-catenin signaling, which resulted in markedly boosted stemness of HCC. It is well-known that CSCs possess strong plasticity of EMT on which tumor metastasis depends greatly [38] . On the other hand, CSCs have the potential of infinite multiplication [39] , [40] . Therefore, the CSCs activation is most likely the underlying cause for HCC oncogenesis and progression (growth and metastasis) induced by the PBOV1 overexpression. Employing the EGFR antibody-mediated endocytosis to improve siRNA delivery efficiency, oncogenesis, tumor growth, and tumor metastasis were effectively suppressed in multiple HCC animal models. Although the great potential of MRI-visible nanomedicine incorporating PBOV1-siRNA as a potent therapeutic agent for HCC treatment was shown, it is worth noting that a toxicity concern exists with PEG–PEI copolymer due to the cationic and nonbiodegradable characters, which may restrict its use in clinic. The main purpose of this study is to demonstrate the oncogenic role of PBOV1 in growth and metastasis of HCC, and our finding may lay a foundation for further developing more applicable siRNA nanomedicines based on biodegradable carriers [41] , [42] . Patient information A total of 286 paraffin-embedded, archived HCC samples, which were histopathologically and clinically diagnosed by the Department of Pathology, First Affiliated Hospital of Sun Yat-sen University from 2002 to 2010. All patients were older than 18 years of age with complete clinical and laboratory data. Patients were regularly followed up at the outpatient clinics every 3 months for the first 2 years, every 6 months for the next 3 years, and once annually thereafter. Patients with mixed HCC and cholangiocarcinoma or no follow-up data were excluded. Eight fresh HCC and paired ANT were collected for quantitative RT-PCR, western blotting, and IHC analyses of PBOV1. For the use of these clinical materials and data for research purposes, prior patients’ written consents and approval from the Institutional Research Ethics Committee (IREC) of the First Affiliated Hospital of Sun Yat-sen University were obtained, in accordance with the rules and regulations concerning ethical issues on research use of human subjects in China. The study protocol conformed to the ethical guidelines of the current Declaration of Helsinki was approved by the IREC of the First Affiliated Hospital of Sun Yat-sen University. Clinical information was summarized in Supplementary Table 1 . RT-PCR assay Total RNA from cells and surgically obtained fresh tumor tissues and their adjacent noncancerous tissues were extracted using the Trizol reagent (Invitrogen) according to the manufacturer’s instruction. The extracted RNA was pretreated with RNase-free DNAse, and 2 μg of RNA from each sample was used for cDNA synthesis. The qRT-PCR primers to amplify PBOV1 were: forward, 5′-TTTGGATAAGTAGAGAAGAC-3′; reverse, 5′-AAGGAACCAGAAATATGAGG A-3′. The control β-actin primers were: forward, 5′-ATTCCACCCATGGCAAATTC-3′; reverse, 5′-ATTCCACCCATGGCAAATTC-3′. qRT-PCR was carried out using the FastStart Universal SYBR Green Master (Roche, Toronto, ON, Canada) on the Bio-Rad CFX96 qRT-PCR detection system (Bio-Rad Laboratories, Hercules, CA, USA). Expression data were normalized to the geometric mean of housekeeping gene β-actin to control the variability in expression levels as described in literatures. Western blotting assay Cells or tissues were lysed for total protein extraction in radioimmunoprecipitation assay buffer (50 mM Tris-HCl, pH 7.4, 150 mM NaCl, 1% NP-40, 0.25% Na-deoxycholate, 1 mM EDTA, and 1 mM NaF) together with a protease inhibitor cocktail (Sigma-Aldrich, St. Louis, MO). Proteins were separated by 10% sodium dodecyl sulphate-polyacrylamide gel electrophoresis and transferred to polyvinylidene difluoride membranes (Amersham Life Science, Piscataway, NJ). Membranes were incubated for 1 h in a blocking buffer containing 5% nonfat dry milk and then probed with indicated antibodies. Bound primary antibodies were then probed with respective secondary antibodies labeled with horseradish peroxidase. Immunolabeled proteins were detected using the ECL system (Amersham Life Science, Piscataway, NJ). Band intensities were quantified using NIH ImageJ software. The membranes were then stripped and reprobed with an anti-β-actin antibody as a loading control. 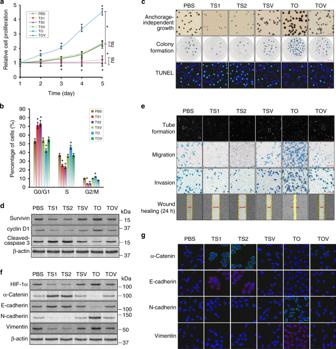Fig. 3 The relationship between PBOV1 expression level and Hep3B cell growth/metastasis property in vitro.aHep3B cell growth rates determined by MTT assay.bHep3B cell cycle analysis by flow cytometry assay.cCell proliferation reflected by anchorage-independent growth assay (first panel, top down; Scale bar, 1 mm), cell colony formation assay (second panel, top down; Scale bar, 10 mm), and terminal deoxynucleotidyl transferase-mediated dUTP nick end labeling assay (TUNEL) cell apoptosis assay (third panel, top down; Scale bar, 20 μm) (assay; Blue, DAPI-indicating nuclei; green, FITC indicating apoptotic nuclei).dProtein expression levels of survivin, cyclin D1, and cleaved-caspase 3 determined by western blotting assay.eTube formation assay by human liver tumor endothelial cells (SK-Hep1) cultured on Matrigel-coated plates with conditioned media collected from the Hep3B cell incubation (first panel, top down; Scale bar, 100 μm). Hep3B cell migration ability determined by transwell migration assay (second panel, top down; Scale bar, 50 μm). Hep3B cell invasion ability determined by transwell invasion assay (third panel, top down; Scale bar, 50 μm). Hep3B cell mobility measured by testing the rate of wound healing at 24 h after serum starvation and wound creation (fourth panel, top down; Scale bar, 500 μm) (See also Supplementary Fig.5b).fProtein expression levels of angiogenesis marker HIF-1α, epithelial markers α-Catenin and E-cadherin, and mesenchymal markers N-cadherin and Vimentin determined by western blotting assay.gImmunofluorescence assays for epithelial markers α-Catenin and E-cadherin, and mesenchymal markers N-cadherin and Vimentin. Scale bar, 20 μm (Blue, DAPI-indicating nuclei; green, FITC indicating α-Catenin or N-cadherin protein; red, Cy5 indicating E-cadherin or Vimentin protein). (See also Supplementary Fig.5d). Data were represented as means ± S.D. Error bars represent the S.D. values (n= 3;*P<0.05; ns, not significant. Significant differences were analyzed by two-way ANOVA with multiple comparisons for (a); Student’sttest for (a) and (b), compared with PBS control group) Information and dilution of antibodies used in this study were listed in Supplementary Table 3 . Full images of the blots are provided in Supplementary Fig. 13 . All the experiments were independently performed three times as the least. IHC analysis IHC analysis was conducted to study altered protein expression in paraffin-embedded human HCC samples. Information and dilution of antibodies used in this study are listed in Supplementary Table 3 . Immunostaining was reviewed and scored independently by three observers based on the proportion of positively stained tumor cells and intensity of staining. Tumor cell proportion was scored as follows: 0 (no positive tumor cells), 1 (35% positive tumor cells), 2 (35–70% positive tumor cells), and 3 (>70% positive tumor cells). Staining intensity was graded according to the following criteria: 0 (no staining), 1 (weak staining: light yellow), 2 (moderate staining: yellow brown), and 3 (strong staining: brown). Staining index was calculated as: staining intensity score × the proportion score of positive tumor cells. PBOV1 expressions were evaluated according to the staining index, with scores of 0–4, 6, or 9. The cutoff value 3.5 for high and low expression levels were chosen in heterogeneity analysis for the log-rank test of overall and DFSs. That is, staining index >3.5 represents high PBOV1 expression, whereas staining index <3.5 indicates low PBOV1 expression. Plasmids pMSCV/PBOV1 overexpressing human PBOV1 plasmid (PBOV1-pDNA) was generated by subcloning the PCR-amplified human PBOV1 coding sequence into pMSCV vector (pDNA-vector). To silence endogenous PBOV1, two shRNA oligonucleotides were cloned into the pSuper-retro-puro vector (psiRNA-vector) to generate pSuper-retro-PBOV1-siRNAs (PBOV1-psiRNA). The sequences of two siRNAs were as follows: 5′-GCAGACACACTTGACCATGAA-3 for PBOV1-psiRNA1 and 5′-CCAGCCAAGTAACTGAACCAT-3′ for PBOV1-psiRNA2. PBOV1 shRNA was synthesized by Shanghai Genepharma. Nanocarrier preparation PEI (MW = 25 kD), monomethoxy PEG (mPEG-OH, MW = 2 kD), succinic anhydride, 2-mercaptoethylamine and dicyclohexylcarbodiimide (DCC), and N-hydroxysuccinimide (NHS) were purchased from Sigma-Aldrich (St Louis, MO, USA). For the synthesis of mPEG-g-PEI, mPEG-OH (4.0 g) was vacuum dried and dissolved in 30 mL anhydrous THF. After the above solution was dropwise added to 20 mL of anhydrous THF solution containing 3.2 g N,N’-carbonyldiimidazole (CDI), the mixture was stirred overnight under argon. A total of 200 μL of distilled water was added to terminate the reaction. After the solution was mixed with a large amount of cold diethyl ether, the precipitate was collected by filtration and vacuum dried at room temperature to get CDI-activated mPEG (mPEG-CDI). PEI (1.1 g) and mPEG-CDI (0.8 g) were dissolved in 20 mL chloroform. The mixture was stirred at room temperature for 24 h and then dialyzed against chloroform (MWCO = 3.5 kDa). After partial solvent was evaporated under reduced pressure, the concentrated solution was added into a large amount of cold diethyl ether. The precipitate was collected by filtration and dried in vacuum at room temperature. For the synthesis of MAL-PEG-OH, HO-PEG-NH 2 (Mn = 3.6 kD, 3.0 g) was dissolved in 15 mL saturated aqueous solution of NaHCO 3 , and then the mixture was cooled to 0 °C. After N-methoxycarbonylmaleimide (0.42 g) was added, the solution was stirred for 10 min. A total of 30 mL water was added and the solution was stirred for 45 min. The pH value of the solution was adjusted to 3.0 with 0.5 M sulfuric acid, and then the mixture was extracted with CH 2 Cl 2 and dried with Na 2 SO 4 . After filtering off Na 2 SO 4 , the solution was added to a large amount of cold diethyl ether. The precipitate was collected by filtration and vacuum dried to a constant weight at room temperature. For SPION encapsulation with PEG-g-PEI, PEG-g-PEI (300 mg) was dissolved in 3 mL of chloroform, and then SPION (15 mg) was dispersed into the above solution. The reaction mixture was stirred overnight at room temperature and then precipitated into large amount of hexane. The precipitate was collected by centrifugation, washed with hexane, and vacuum dried to remove the organic solvents. The product thus prepared was dispersed into distilled water under sonication and filtered through a 220-nm membrane to remove large aggregates. For the synthesis of final scAb-conjugated magnetic nanocarrier [43] , 10 μL of EGFR antibody in aqueous solution (1 μg/μL) was dissolved in a mixture of 40 μL PBS (pH 7.4) and 10 μL EDTA aqueous solution (0.5 M). A 500 μL PBS containing 2-mercaptoethylamine (60 mg) and 10 μL EDTA solution (0.5 M) was mixed with the antibody solution. After incubation for 90 min at 37 °C, the obtained scAb solution was purified by ultrafiltration in an Amicon cell (MWCO = 5 kD) and washed times times with PBS (pH 7.4, each 500 μL containing 10 μL of 0.5 M EDTA solution). A total of 10 μg of MAL-PEG-COOH dissolved in 10 μL PBS containing 10 μL of 0.5 M EDTA solution was added to the scAb solution and then incubated overnight at 4 °C. The resultant solution containing scAb functionalized PEG (scAb-EGFR-PEG-COOH) was washed three times with PBS (pH 7.4) using ultrafiltration in an Amicon cell (MWCO = 5 kD). After DCC (5 μg), NHS (5 μg) and PEG-g-PEI-SPION (10 μg) were added, the solution was adjusted to 100 μL with PBS, and incubated overnight at 4 °C. Polyplex formation pDNA or psiRNA plasmid (4 mg) and an appropriate amount of nanoparticle were dissolved separately in 0.9% sodium chloride solution. The two solutions were mixed by vigorous pipetting and then kept at room temperature for 60 min to allow polyplex formation. The amount of delivery agent (nontargeted PEG-g-PEI-SPION or scAb-EGFR-PEG-g-PEI-SPION) to complex the plasmid (PBOV1-pDNA or PBOV1-psiRNA) was based on the designed experimental N/P ratios, which were calculated as the number of nitrogen atoms in delivery agents over that of the phosphate groups in plasmids. Determination of plasmid complexation Gel electrophoresis was performed on a Bio-Rad Sub-Cell electrophoresis cell (Bio-Rad Laboratories, Inc., USA), and images were obtained on a DNR Bio-Imaging Systems (DNR Bio-Imaging Systems Ltd., Israel). Complex formation was induced at various N/P ratios in a final volume of 6× agarose gel loading dye mixture (i.e., 10 μL). The appropriate amount of delivery agent and plasmid were dissolved separately in a neutral aqueous solution containing 0.9% sodium chloride. The two solutions were mixed by vigorous pipetting, loaded onto the 0.9% agarose gels with ethidium bromide (0.1 μg/ml), and ran with tris–acetate buffer at 100 V for 40 min. Plasmid band shifts were revealed by irradiation with UV light. Zeta potential and size measurements The hydrodynamic sizes and zeta potentials of scAb-EGFR-PEG-g-PEI-SPION/plasmid particles were determined by DLS measurements. Zeta potential measurement of nanoparticles was carried out in the standard capillary electrophoresis cells, using a ZetaPlus instrument (Brookhaven, NY, USA) at a position of 45° angle at 25 °C. The average values plus standard deviations were based on the data of five runs. Nanoparticle size was determined on the same instrument at 25 °C. Scattering light was detected at 90° angle, and the sizes given are the means of five runs plus standard deviations. Cell culture HCC cell lines Hep3B, SNU423, PLC/PRF/5, and HEPG2/2.2.1, hepatoblastoma cell line HepG2, and HCC endothelial cell line SK-Hep1 were obtained from ATCC (Manassas, VA, USA). HCC cell lines HLE and HLF were obtained from the Japanese Collection of Research Bioresources Cell Bank (JCRB Cell Bank, Japan). HCC cell lines SMMC-7721, Huh7, and BEL7402 and human hepatocyte L02 and HHL-5 were obtained from Shanghai Cell Bank of Chinese Academy of Science (Shanghai, China). All cell lines used were authenticated and confirmed to be mycoplasma negative by MycoAlert TM Mycoplasma Detection Kit (Lonza, Basel, Switzerland). Human hepatocytes (L02 and HHL-5) and human HCC cell lines (Hep3B, BEL7402, SNU423, SMMC-7721, PLC/PRF/5, Huh7, HLE, HLF, and HepG2.2.1), HCC endothelial cell line (SK-Hep1), and hepatoblastoma cell line (HepG2) were cultured in the DMEM medium (Invitrogen, Carlsbad, CA, USA) supplemented with 10% FBS (HyClone, Logan, UT, USA) in a humidified atmosphere of 5% CO 2 at 37 °C. Three cell lines including Hep3B, BEL7402, and SMMC-7721 underwent the PBOV1 gene regulation experiments. Each of the cell line was grouped for culture with PBS or different nanocomplexes as follows: scAb-EGFR-PEG-g-PEI-SPION/PBOV1-psiRNA1 (TS1 group), scAb-EGFR-PEG-g-PEI-SPION/PBOV1-psiRNA2 (TS2 group), scAb-EGFR-PEG-g-PEI-SPION/psiRNA-vector (TSV group), scAb-EGFR-PEG-g-PEI-SPION/PBOV1-pDNA (TO group), scAb-EGFR-PEG-g-PEI-SPION/pDNA-vector (TOV group), nontargeted PEG-g-PEI-SPION/PBOV1-psiRNA1 (NS1 group), nontargeted PEG-g-PEI-SPION/PBOV1-psiRNA2 (NS2 group), nontargeted PEG-g-PEI-SPION/psiRNA-vector (NSV group), nontargeted PEG-g-PEI-SPION/PBOV1-pDNA (NO group), nontargeted PEG-g-PEI-SPION/pDNA-vector (NOV group), 1 mmol/L free EGFR-IgG competitive inhibition + scAb-EGFR-PEG-g-PEI-SPION/psiRNA-vector group (CTS group), or PBS (PBS group). The plasmid mass in all nanomedicines TS1, TS2, TSV, TO, TOV, NS1, NS2, NSV, NO, and NOV groups was set to 0.5 μg/mL in cell culture medium. Cell uptake of polyplexes assessed by MRI A total of 1 × 10 6 of Hep3B cells were washed and trypsinized after incubation with scAb-EGFR-PEG-g-PEI-SPION/psiRNA-vector (TSV group) or nontargeted PEG-g-PEI-SPION/psiRNA-vector (NSV group) at Fe concentrations of 5, 10, 20, 40, and 80 μg/mL in an EGFR antibody-free DMEM medium for 0.5 h. For the free-ligand competition experiment, cells were pretreated with 1 mmol/L EGFR-IgG antibody for 30 min before incubation with scAb-EGFR-PEG-g-PEI-SPION/psiRNA-vector at various Fe concentrations (CTS group). Cells were then collected and scanned under a 1.5-T MRI scanner (Intera; Philips Medical Systems, Best, The Netherlands) at room temperature. A circular surface coil with an inner diameter of 11 cm was used. T2-weighted images were acquired using the following parameters: TR/TE, 5,000/100 ms; FOV, 150 mm; matrix, 256 × 256; and slice thickness, 1.5 mm. The MRI T2 signal intensities within the region of interest were measured. Fluorescence study on cellular uptake of nanomedicines To enable confocal laser scanning microscopic (CLSM) observation of the cells after incubation, the delivery agent scAb-EGFR-PEG-g-PEI-SPION, or nontargeted PEG-g-PEI-SPION were labeled with Oregon Green 488 and POPO-3 according to the manufacturer’s protocols (in TSV group or NSV group, respectively). The POPO-3 labeled psiRNA-vector was complexed with the Oregon Green-labeled delivery agent at N/P = 10. Hep3B cells were seeded at a density of 5 × 10 5 cells per well in six-well plates. The formed polyplex (Fe concentration: 20 μg/mL) was then added into EGFR antibody-free culture medium for cell culture. For a free-ligand competition experiment (CTS group), cells were pretreated with 1 mmol/L free EGFR antibody for 0.5 h before incubation with fluorescence-labeled scAb-EGFR-PEG-g-PEI-SPION/psiRNA-vector. After 0.5 h, cells were washed three times with fresh PBS, fixed, and further incubated with DAPI for nuclei staining. CLSM observation was carried out on a Zeiss LSM 510 META microscope as described (Carl Zeiss Co., Ltd., Gottingen, Germany). Prussian blue staining for cell uptake of polyplexes Hep3B cells at a density of 5 × 10 5 cells per dish were incubated for 0.5 h in complete medium added with polyplex. Then, cells were washed with PBS for three times, fixed with 4% glutaraldehyde for 10 min, and incubated at 37 °C with 2 mL Prussian blue solution comprising equal volumes of 2% hydrochloric acid aqueous solution and 2% potassium ferrocyanide trihydrate for 30 min. After treatment with 0.5% neutral red for 3 min, the iron staining was finally observed using optical microscope. For in vivo study, full-thickness histological sections of tumors were collected at 6 h after injection for analysis of tumor Fe accumulation using Prussian blue staining. MTT assay Hep3B, SMMC-7721, and BEL7402 cells were seeded in 96-well plates at the density of 1 × 10 3 cells per well and incubated overnight. Next day, 50 ng of each plasmids were transfected into cells and incubate for another 24 h. Then, 150 μL of growth medium was replaced into each well and then 20 μL of MTT solution (5 mg/mL in PBS) was added at each time point. After cells were further incubated for 4 h, the supernatant in the wells was discarded and 150 μL of DMSO was added to dissolve the substrate for 10 min. After gentle agitation for 5 min, the absorbance at 570 nm in each well was recorded on a Tecan Infinite F200 Multimode plate reader. Flow cytometry cell cycle analysis The effect of polyplexes on cell cycle of Hep3B cells as an example was evaluated by propidium iodide staining and flow cytometry assays. The cells were harvested 48 h after incubation in complete medium, washed with PBS and fixed in 70% cold ethanol for 1 h. RNA was digested by incubating the samples with 1 mg/mL RNase A (Invitrogen, Carlsbad, CA) for 30 min at 37 °C. Propidium iodide (50 μg/mL, Sigma-Aldrich, St. Louis, MO) was then added and the samples were recorded using the Navios Flow Cytometers (Beckman Coulter, Miami, FL). Cell cycle analysis was performed using the multi-cycle analysis software (Phoenix Flow Systems, San Diego, California). Experiments were conducted in triplicate to obtain the averaged values and standard deviation. Anchorage-independent growth ability assay Hep3B cells were treated with complete medium containing polyplex for 48 h, trypsinized and suspended in 2 mL (500 cells for each well) of complete medium added with a polyplex plus 0.3% agar (Sigma). The above mixture was plated on a gel layer consisting of complete medium and 1% agar, and then covered with a gel layer consisting of complete medium and 0.3% agar. After 10 days incubation at 37 °C in 5% CO 2 atmosphere, viable colonies larger than 0.1 mm in diameter were counted. For each group of the cell line, the experiment was performed in triplicate for at least three times. Colony formation assay Hep3B cells were treated with complete medium containing polyplex for 48 h. The cells were trypsinized, plated on 6-well plates (200 cells each well) and then cultured in medium containing polyplex with 10 % FBS for 2 weeks. The colonies were fixed with 4% paraformaldehyde for 5 min and stained with 1% crystal violet for 30 s. Colonies of more than 50 cells were counted. For each group of the cell line, the experiment was performed in triplicate for at least three times. In vitro TUNEL assay Hep3B cell apoptosis was measured using TUNEL assay. Hep3B cells were plated at the density of 1 × 10 3 cells/well in six-well plates and then incubated with complete medium for 24 h, which was followed by polyplex treatment and then another 24 h incubation at 37 °C in 5% CO 2 atmosphere. The numbers of living cells were determined by trypan blue exclusion. The DeadEnd Fluorometric TUNEL System (Promega,Madison, WI) and ApopNexinTM Fluorescein Isothiocyanate Apoptosis Detection Kit (Millipore, Lake Placid, NY) were employed for the evaluation of cell apoptosis. The images were captured on a fluorescence microscope equipped with a digital camera. The percentage of apoptotic cells was obtained upon counting TUNEL-positive cells. For each group of the cell line, the experiment was performed independently in triplicate. Tube formation assay Approximately human Hep3B cells (1 × 10 5 per well) was incubated in polyplex-containing DMEM medium for 72 h on the 24-well plates at 37 °C in a humidified atmosphere of 5% CO 2 . The plasmid mass for each well was set to 0.05 μg. The medium in each well was replaced with fresh DMEM medium free of polyplex to further incubate the cells for 24 h. Matrigel (200 μL) was pipetted into each well of 24-well plates and polymerized for 30 min at 37 °C. Finally, culture medium having been used for Hep3B incubation was withdrawn for incubating the human HCC endothelial cells (SK-Hep1 cells) for 24 h at 37 °C in 5% CO 2 atmosphere. SK-Hep1 cells activated by the Hep3B culture medium, were seeded on matrigel at a density of 1 × 10 4 cells per well on 24-well plate. 200 μL of medium from Hep3B incubation was added into each well. Pictures were taken under a 100× bright-field microscope and capillary tube formation was counted in five random fields. For each group of the cell line, the experiment was performed independently for three times. Boyden chamber migration and invasion assay Hep3B cells were treated with complete medium containing polyplex for 48 h. Next, cells were seeded into the 8 μm pore inserts with (invasion assay) or without (migration assay) the coating of 50 μL Matrigel (2 × 10 4 cells each pore). After 24 h, the cells that passed through the filter to arrive the lower chamber were fixed with 1% paraformaldehyde, stained with hematoxylin and counted (10 random 100 fields per well). For each group of the cell line, the experiment was performed independently for three times. Wound-healing assay Hep3B cells were seeded in six-well plates, incubated with complete medium containing polyplex until reaching 90% confluence. Cells were then serum-starved for 24 h, and then a linear wound was created in the confluent monolayer using a pipette tip. Wounds were observed and photographed immediately as the time point 0 h, and thereafter at the time points 12 and 24 h. For each group of the cell line, the experiment was performed independently for three times. Sphere formation assay Hep3B cells were treated for 48 h with complete medium containing polyplex. Cells were trypsinized and washed twice with PBS. Next, cells were seeded at 1 × 10 3 cells/well in the six-well ultralow attachment plates. Cells were cultured for 14 days in DMEM/F-12 with 2% B-27 supplement culture medium supplemented with 10 ng/mL human recombinant basic fibroblast growth factor (PeproTech Inc, Rocky Hill, NJ, USA), 10 ng/mL epidermal growth factor (PeproTech) and 0.5 μg/mL plasmid nanoparticle mass. Afterwards, spheres were photographed and counted. For each group, the experiment was performed independently for three times. Fluorescence microscopy assay Cells were trypsinized, seeded on coverslips (Thermo Fisher Scientific, Lafayette, CO) and incubated overnight. The cells were then washed with PBS and fixed with 4% paraformaldehyde for 1 min and then with prechilled methanol for another 15 min at room temperature. Next, cells were permeabilized with 0.2% Triton X-100 in PBS (PBS-T) for 15 min, blocked with 10% BSA in PBS-T for 30 min, and incubated with primary antibodies overnight at 4 °C. Cells were then incubated with species-specific Cy5- or fluorescein Isothiocyanate (FITC)-conjugated secondary antibody (Jackson Immuno-Research Laboratories) for 1 h at room temperature. Coverslips were mounted with ProLong Diamond Anti-fade reagent with DAPI (Invitrogen). Gray level images were acquired under a Zeiss Axio Imager.Z2 microscopeor Zeiss LSM 700 confocal microscope. Proportion of CSCs assay CSCs proportion was measured by flow cytometer analysis of the ratio of side population cells, which was attributed as CSCs. Hep3B cells were treated with complete medium containing polyplex for 48 h. Suspensions were labeled with Hoechst 33342 dye (Sigma‑Aldrich, St. Louis, MO, USA). Cells were resuspended in pre-warmed high-glucose DMEM containing 10% FBS (1 × 10 6 cells/mL), and then were incubated at 37 °C for 90 min with intermittent shaking. At the end of the incubation, the cells were washed with ice-cooled PBS, centrifuged at 4 °C, and resuspended in ice-cooled HBSS containing 2% FBS in the dark. The Hoechst 33342 dye was excited at 357 nm and its fluorescence was analyzed by dual-wavelength measurements (blue, 402–446 nm; red, 650–670 nm). For CD133 + /EpCAM + cell analyses, cells after treatment were washed, resuspended, and then incubated at 4 °C in the dark for 40 min with fluorescence-labeled antibodies against human CD133-PE and EpCAM-PerCP/Cy5.5, and their isotype IgG at concentrations recommended by the manufacturer. The samples were analyzed on a FACS Aria III flow cytometer (BD Biosciences). Information and dilution of antibodies used in this study were listed in Supplementary Table 3 .The results were analyzed using FlowJo software (Ashland, OR, USA). All FACS plots in our results have their corresponding negative controls. Luciferase reporter assay Luciferase assay were performed as described. 2 × 10 4 cells were seeded in triplicate in 48-well plates and allowed to settle for overnight. Cells were transfected with 300 ng of β-catenin luciferase reporter plasmid or the control-luciferase plasmid plus 5 ng of pRL-TK Renilla plasmid (Promega) using the Lipofectamine 2000 reagent, following the manufacturer’s recommendation. Luciferase and Renilla signals were measured 48 h after transfection using the Dual Luciferase Reporter Assay Kit (Promega) according to the manufacturer protocol. Establishment and treatment of tumor models Male BALB/c-nu nude mice (4 weeks old) were purchased from Vital River Laboratories (Beijing, China), housed in specific pathogen-free facilities and maintained in 12 h light/12 h dark cycles with free access to food and water. All experimental procedures involving animals were in accordance with the Guide for the Care and Use of Laboratory Animals (NIH publication nos. 80–23, revised 1996) and followed the institutional ethical guidelines for animal experiments. All animal experimental procedures were approved by the Institutional Animal Care and Use Committee (IACUC) of the First Affiliated Hospital of Sun Yat-sen University. The retention and use of animals were in compliance with national and local laws and regulations. For the liver orthotropic moldel, 1 × 10 6 Hep3B, SMMC-7721 or BEL7402 cells in 200 μl of culture medium were injected into the right lobe of liver of male BALB/c-nu nude mice. For the intrahepatic orthotropic model, tumor weight was monitored after 30 days of treatment. When the tumor volume reached about 100 mm 3 , mice were subjected to in vivo MRI and fluorescence imaging for cellular uptake or diagnostic assay. To assess the tumor incidence and growth rates in subcutaneous transplantation tumor model, different amounts of Hep3B cells (1 × 10 3 , 1 × 10 4 , 1 × 10 5 , or 1 × 10 6 ) in 200 μL of culture medium were injected into the dorsal right flank of nude mice. Tumor growth of subcutaneous tumor was monitored once every 3 days. Length (L) and width (W) measurements were obtained with calipers, and tumor volumes were calculated using the equation (L × W 2 )/2. 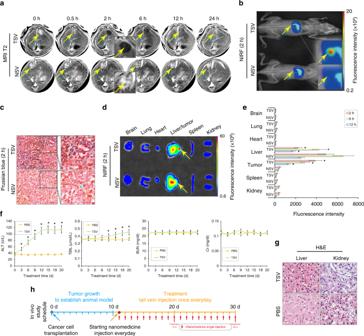Fig. 4 In vivo biodistribution and toxicological study of theranostical nanomedicine in Hep3B liver orthotropic model.aT2-weighted MRI examination showing a nonlinear change in tumor signal intensity against tracing time (0, 0.5, 2, 6, 12, and 24 h after tail vein single injection). Yellow arrows indicate the location of the tumor.bNear-infrared fluorescence (NIRF) imaging of mice 2 h after nanomedicine single injection. The fluorescent reporter used for NIRF was Alexa Fluor 750. Yellow arrows indicate the location of the tumor (See also Supplementary Fig.10).cPrussian blue staining performed on histological sections of orthotropic tumors 2 h after single injection. Scale bar, 100 μm.dNIRF images of various mice organs harvested 2 h after nanomedicine single injection (see also Supplementary Fig.10).eAveraged fluorescence intensities of mice tumors and major organs at 2, 6, and 12 h after a single injection of nanomedicine.fSerum liver function markers alanine transaminase (ALT)/total bilirubin (TBIL) and renal function markers blood urea nitrogen (BUN)/creatinine (Cr) were assessed during the period from 0 to 20 days after namomedicine injection once a day under therapeutic dosage (plasmid dose 8 μg).gHaematoxylin and eosin (H&E) staining of the liver and kidney tissues from mice after 20 days of treatment for evaluations of tissue inflammation and structural damage. Scale bar, 20 μm. (nanomedicine injected once a day at plasmid dose 8 μg).hSchedule illustration of in vivo study. Data were represented as means ± S.D. Error bars represent the S.D. values (n= 12,*P< 0.05, Student’sttest, compared with NSV group or PBS control group). For the pulmonary metastatic tumor model, the Hep3B cells (5 × 10 6 per mouse) were injected intravenously into the tail vein of mice. Four weeks later, the mice were killed and the lungs were removed, fixed with 3.7% formaldehyde and sectioned. The number of mice having pulmonary metastasis was determined. On the tenth day after cancer cell implanted, the tumor-bearing mice of each model were randomly divided into various therapeutic groups ( n = 12), and therapy was conducted with different injections as follows: scAb-EGFR-PEG-g-PEI-SPION/PBOV1-psiRNA1 (TS1 group), scAb-EGFR-PEG-g-PEI-SPION/PBOV1-psiRNA2 (TS2 group), scAb-EGFR-PEG-g-PEI-SPION/psiRNA-vector (TSV group), scAb-EGFR-PEG-g-PEI-SPION/PBOV1-pDNA (TO group), scAb-EGFR-PEG-g-PEI-SPION/pDNA-vector (TOV group), nontargeted PEG-g-PEI-SPION/PBOV1-psiRNA1 (NS1 group), nontargeted PEG-g-PEI-SPION/PBOV1-psiRNA2 (NS2 group), nontargeted PEG-g-PEI-SPION/psiRNA-vector (NSV group), nontargeted PEG-g-PEI-SPION/PBOV1-pDNA (NO group), nontargeted PEG-g-PEI-SPION/pDNA-vector (NOV group) or the same volume of neat PBS (PBS group). Different nanomedicines with the same Fe concentration and plasmid dose were injected into the tail vein of the tumor-bearing mice ( n = 12). Nanomedicine dissolved in 150 μL of PBS was injected once every day at a dose of 8 μg plasmid via the tail vein of the tumor-bearing mice. After 20 days of treatment, animals were sacrificed and tumors were harvested, weighed, and paraffin embedded. For in vivo BrdU assay, the mice were i.p. injected with 50 mg/kg BrdU (about 1 mg) 24 h before sacrificed. Serial 5.0 μm sections of tumor specimens were cut and subjected to IHC staining, MVD staining and in vivo TUNEL assays. Experiments were performed independently at least three times. In vivo MRI scan of cellular uptake of polyplexes At different time points after polyplex injection, the in vivo distribution of SPION was detected by MRI scan using a clinical 1.5-T system (Intera; Philips Medical Systems, Best, the Netherlands) with a 50-mm linearly polarized birdcage radiofrequency mouse coil (Chenguang Medical Technologies Co., Shanghai, China). Axial abdominal images were obtained using a two-dimensional turbo spin-echo T2-weighted sequence (TR/TE = 2600/100 ms; flip angle = 90°; NSA = 6) and a two-dimensional turbo spin-echo T1-weighted sequence (TR/TE = 300/17 ms; flip angle = 120°; NSA = 6). The other parameters for these sequences were as follows: FOV = 40 mm, matrix = 256 × 256, section thickness = 1.0 mm, and no intersection gap. NIRF imaging The polyplexes and amine-reactive Alexa Fluor 750 dye were dissolved in 0.1 M sodium bicarbonate buffer (0.5 mg/mL) and DMSO (10 mg/mL), respectively. Then, the polyplex solution was mixed with dye solution at a volume ratio of 1:10. The reaction was conducted for 1 h at room temperature under magnetic stirring. The unconjugated dye was eliminated from the solution by ultrafiltration in an Amicon cell (regenerated cellulose membrane, MWCO = 5 kDa). Then, the polyplex solution was washed several times with PBS (pH 7.4) until no fluorescence absorption of Alexa Fluor 750 was detectable in the filtrate. Before imaging study, the mice were anesthetized by intraperitoneal injection of 150 mL 4% chloralic hydras. Optical imaging was performed using an in vivo fluorescence imaging system (Carestream, USA) with emission at 720 nm and excitation at 790 nm after the mice were injected with the polyplex solutions. The fluorescence images were captured at different time points. The fluorescence intensity was quantified using Carestream MI software. Ex vivo imaging study of major organs and tumors were performed as well under the same image acquisition conditions. Blood concentrations of siRNA nanomedicines The BALB/c mice were randomly divided into three groups ( n = 6). The Alexa Fluor 750-labeled NSV, TSV, and PBS were tail vein injected into the mice of different groups, respectively. The blood samples (150 μL each) were obtained every 2 h after injection. To analyze the blood concentrations of nanomedicines, the fluorescence intensity of Alexa Fluor 750 in the blood was detected by fluorescence spectrophotometer after a 20-fold dilution (Ex: 750 nm; Em: 778 nm). The fluorescence intensities of blood samples at 0 h after injection were employed for data normalization, and the control mice receiving PBS were analyzed for data calibration. In vivo toxicity assay To determine the side effects of polyplexes, mice-bearing tumor were divided randomly into 3 groups ( n = 12 each). Animals received a single injection of 150 μL neat PBS (PBS group), the same volume of PBS containing scAb-EGFR-PEG-g-PEI-SPION/psiRNA-vector at plasmid dose of 8 μg (TSV group), or the same volume of PBS containing scAb-EGFR-PEG-g-PEI-SPION/psiRNA-vector at plasmid dose of 40 μg (5 × TSV group) via the tail vein. 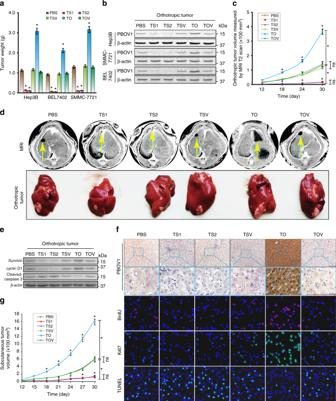Fig. 5 In vivo effects of nanomedicines on proliferation activities in HCC liver orthotropic and subcutaneous models.aTumor weight measured at day 20 after treatment began in Hep3B, SMMC-7721 and BEL7402 liver orthotropic model.bProtein expression levels of PBOV1 determined by western blotting assay in Hep3B, SMMC-7721, and BEL7402 liver orthotropic tumor tissues from mice after treatment for 20 days.cKinetic of the liver orthotropic tumor growth measured by MRI T2 scan at 2 h after nanomedicine injection (nanomedicines injected once every day from day 11; to visulaize the tumors of PBS group by MRI, TOV nanomedicine was injected 2 h before MRI scan).dFirst panel, MRI T2 scan for liver orthotropic tumors; second panel, optical imaging of liver showing orthotropic tumors at day 20 after treatment began.eProtein expression levels of proliferation marker survivin, cell cycle marker cyclin D1 and apoptotic marker cleaved-caspase 3 in Hep3B liver orthotropic tumor tissues at day 20 after treatment began.fFirst and second panel from top down, protein expressions of PBOV1 determined by IHC in liver orthotropic tumors in various treatment groups, and magnified view showing location of PBOV1 expression inside cancer cells (Scale bar, 50 μm); third and fourth panel from top down, in vivo tumor cell proliferation abilities measured by immunofluorescence staining assays for Bromodeoxyuridine (BrdU) and Ki67; fifth panel from top down, tumor apoptosis detected by TUNEL assay (Scale bar, 20 μm) (Blue, DAPI-indicating nuclei; red, Cy5 indicating BrdU location; green, FITC indicating Ki67 protien or apoptotic nuclei).gObservation of the tumor inhibition effect in subcutaneous tumor model during the 20 days of treatment (see also Supplementary Fig.6). Data were represented as means ± S.D. Error bars represent the S.D. values (n= 12;*P< 0.05; ns, not significant. Significant differences were analyzed by two-way ANOVA with multiple comparisons forcandg; Student’sttest for (a,candg), compared with PBS control group) To determine the state of the liver and renal, serum biochemical tests for liver function biomarkers ALT or TBIL and renal function biomarkers BUN or Cr were performed over 72 h after the injection. To further determine the long-term solid organ injury, liver and kidney tissues harvested from mice of TSV, 5 × TSV, or PBS groups after 20 days of treatment were subjected to the H&E staining. In vivo TUNEL assay and immunofluorescence assay Slides were fixed with Histochoice (Amresco). The DeadEnd ™ Fluorometric TUNEL System (Promega, Madison, WI) was used for TUNEL assay according to the manufacturer’s instruction. Nuclei of cells were counterstained with DAPI (Vector Labs). For MVD assay, slides were labeled overnight with primary antibodies. Fluorescent IHC was performed first using monoclonal mouse antihuman anti-CD31 antibody (1:200, Dako), anti-EGFR antibody (1:250, Abcam), anti-BrdU antibody (1:250, Abcam), anti-Ki67 antibody (1:200, Abcam) or isotype control antibodies followed by FITC conjugated goat-anti-mouse IgG (1:1000, Abcam) or Cy5 conjugated goat-anti-mouse IgG (1:1000, Abcam) according to manufacturer’s protocols. The images were analyzed on the BioView Duet fluorescent scanning station using oil objective and DAPI/FITC/Rhodamine single band filters (Semrock). For each piece of the slide, the experiment was performed for three independently times. Coimmunoprecipitation and MS analysis Hep3B cells were transfected with GFP-PBOV1-flag or control empty vector using lipofectamin-2000. After 48 h, cells were lysed in lysis buffer (1% NP-40, 25 nM HEPES, 150 mM NaCl, 1 mM EDTA, 5% Glycerol, pH 7.4) and PBOV1 was immunoprecipitated using anti-FLAG Agarose overnight at 4 °C. The immunoprecipitated material was eluted using FLAG peptide (Sigma-Aldrich). The eluted material was used for western blotting or MS analysis. The MS analysis was performed by BGI (Beijing, China) using the Q-Exactive MS. The detailed data of the mass spectry analysis were described in Supplementary Data 1 and Supplementary Data 2 . 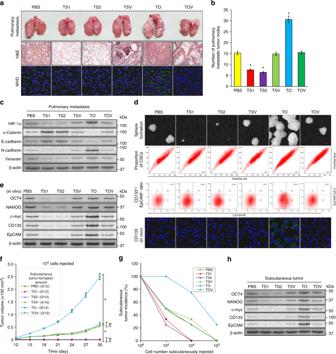Fig. 6 In vivo effects of nanomedicines on metastasis and stemness activities.aPulmonary metastasis (first panel, top down) and H&E staining (second panel, top down; Scale bar, 200 μm) of the metastatic tumor after 20 days of treatment; third panel from top down, tumor angiogenesis determined by microvessel density (MVD) assay (Scale bar, 20 μm; Blue, DAPI-indicating nuclei; green, FITC indicating CD31 protein).bPulmonary metastatic tumor nodes counted after 20 days of treatment.cProtein expression levels of angiogenesis marker HIF-1α, epithelial markers α-Catenin and E-cadherin and mesenchymal markers N-cadherin and Vimentin in pulmonary metastasis tumor tissues.dFirst panel from top down, cell stemness measured by sphere formation assay (Scale bar, 100 μm); second panel from top down, proportions of cancer stem cells (CSCs) measured by Hoechst 33342 dye exclusion assay; third panel from top down, flow cytometry analyses of the percentage of CD133+/ EpCAM+cells in Hep3B cell populations; 4th panel from top down, in vivo CD133+cancer stem cell propotion displayed by immunofluorescence staining (Scale bar, 20 μm; Blue, DAPI-indicating nuclei; green, FITC indicating CD133 protien location).eIn vitro protein expression levels of general stem cell markers (OCT4, NANOG, c-myc) and cancer stem cell surface markers (CD133, EpCAM) determined by western blotting assay.fEffect of nanomedicine treatments on tumor incidence rates and growth speeds in subcutaneous tumor model established via subcutaneous injection of 1 × 104Hep3B cells.gOncogenic potential determined by limiting dilution assay to measure tumor incidence; various amounts of Hep3B cells (1 × 103, 1 × 104, 1 × 105or 1 × 106) were injected subcutaneously before nanomedicine treatment (see also Supplementary Fig.7).hProtein expression levels of stem cell markers and cancer stem cell surface markers in subcutaneous tumor tissues. Data were represented as means ± S.D. Error bars represent the S.D. values (n= 12; *P< 0.05; ns, not significant. Significant differences were analyzed by two-way ANOVA with multiple comparisons for (f); Student’sttest for (b) and (f), compared with PBS control group) 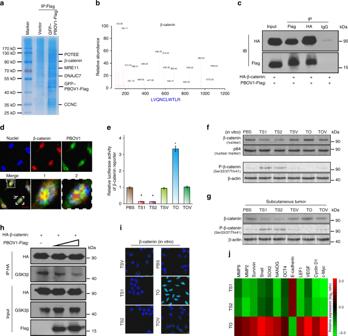Fig. 7 PBOV1 binds to β-catenin and activates Wnt/β-catenin signaling.aRepresentative picture of coomassie blue staining of proteins co-immunoprecipitated with PBOV1.bRepresentative MS plots and sequences of peptides from β-catenin.cImmunoprecipitation assay confirming interaction between PBOV1 and β-catenin.dRepresentative confocal images showing colocalization of PBOV1 and β-catenin (Scale bar, 10 μm).eβ-catenin luciferase-reporter activities analyzed in various groups of Hep3B cells. Data were represented as means ± S.D. Error bars represent the S.D. values (n= 3;*P< 0.05. Significant differences were analyzed by Student’sttest, compared with PBS control group).fProtein expression levels of β-catenin in the nuclear fraction and Phospho-β-catenin (Ser33/37/Thr41) in Hep3B cells in vitro determined by western blotting assay. P84 and β-actin served as loading control.gProtein expression levels of total β-catenin and Phospho-β-Catenin (Ser33/37/Thr41) in Hep3B subcutaneous tumor tissues determined by western blotting assay.hPBOV1 attenuates interactions between β-catenin and GSK-3β in dose-dependent manner.iImmunofluorescence staining of β-catenin in the indicated Hep3B cells. (Scale bar, 20 μm; Blue, DAPI-indicating nuclei; green, FITC indicating β-catenin protein).jReal-time PCR analysis demonstrating an apparent overlap between β-catenin-dependent gene expression and PBOV1-regulated gene expression. The pseudocolour represents the intensity scale for indicated treatment groups versus PBS control group, calculated by log2transformation Statistical analysis The data are expressed as the means ± standard deviation (S.D.). The χ 2 test and Fisher’s exact test were used to analyze the relationship between PBOV1 expression and the clinicopathological characteristics. Survival curves were plotted by the Kaplan–Meier method and were compared using the log-rank test. Survival data were evaluated using univariate and multivariate Cox regression analyses. Experimental data were analyzed by Student’s t tests for two groups and two-way analysis of variance for multiple groups. A value of P < 0.05 was considered statistically significant. All statistical tests were performed using SPSS software (version 13.0, SPSS Inc.). Data availability The authors declare that all the data generated or analyzed during this study and supporting the findings of this study are included in the article and its Supplementary Information files or available from the corresponding author upon reasonable request.